Molecular and clinical determinants of response and resistance to rucaparib for recurrent ovarian cancer treatment in ARIEL2 (Parts 1 and 2) ARIEL2 (NCT01891344) is a single-arm, open-label phase 2 study of the PARP inhibitor (PARPi) rucaparib in relapsed high-grade ovarian carcinoma. In this post hoc exploratory biomarker analysis of pre- and post-platinum ARIEL2 samples, RAD51C and RAD51D mutations and high-level BRCA1 promoter methylation predict response to rucaparib, similar to BRCA1 / BRCA2 mutations. BRCA1 methylation loss may be a major cross-resistance mechanism to platinum and PARPi. Genomic scars associated with homologous recombination deficiency are irreversible, persisting even as platinum resistance develops, and therefore are predictive of rucaparib response only in platinum-sensitive disease. The RAS, AKT, and cell cycle pathways may be additional modulators of PARPi sensitivity. Rucaparib is an inhibitor of poly(ADP-ribose) polymerase (PARP) 1, PARP2, and PARP3, DNA damage repair enzymes in the base excision repair pathway [1] . Homologous recombination deficiency (HRD) sensitizes neoplasms to rucaparib and other DNA-damaging agents (e.g., platinum-based chemotherapy) [2] , [3] , and platinum sensitivity in high-grade ovarian carcinoma (HGOC) is a strong clinical predictor of benefit from PARP inhibitors (PARPi) [4] , [5] , [6] , [7] . Genetic, epigenetic, and genomic biomarkers can suggest the presence of HRD and help identify patients most likely to respond to PARPi [8] , [9] , [10] . Germline and somatic BRCA1 or BRCA2 ( BRCA ) mutations are well-defined biomarkers for PARPi response for a number of cancer types, including breast, ovarian, pancreatic, and prostate [11] , [12] , [13] , [14] , [15] , [16] . Alterations in other homologous recombination repair (HRR) pathway genes, including PALB2 , RAD51C , and RAD51D , have been associated with improved responses to rucaparib and other PARPi [17] , [18] , [19] . However, the extent to which many HRR genes contribute to PARPi sensitivity remains unclear [20] . BRCA1 and RAD51C promoter methylation results in transcriptional silencing [21] and commonly leads to HRD in HGOC [22] . In preclinical studies, BRCA1 or RAD51C methylation led to increased sensitivity to PARPi and platinum [23] , [24] , [25] , but establishing a consistent association of methylation with clinical responses has been elusive [26] , [27] . Given the variety of mechanisms that can result in HRD, methods for identifying HRD cancers independent of the mechanisms involved are desirable. HRD cancers exhibit high genomic instability, characterized by deletions of large genomic segments (genome-wide loss of heterozygosity [LOH]), among other genomic aberrations [28] , [29] . Next-generation sequencing (NGS) can identify multiple patterns of genomic change, including copy number variations, single-nucleotide variations, insertions/deletions, rearrangements characteristic of HRD [29] , [30] , and others [31] , [32] , [33] , [34] . HGOCs with a BRCA mutation or BRCA1/RAD51C methylation have high levels of genomic LOH [25] . Patients with BRCA wild-type ( BRCA wt) HGOC with high LOH (≥16%) show greater clinical benefit from rucaparib than those with low LOH [7] . High LOH is also correlated with improved response to platinum and other PARPi [6] , [35] . However, genomic scars accumulate in HRD cancer cells over time and do not disappear when HRR is restored or other PARPi resistance mechanisms develop, making them imperfect biomarkers of PARPi sensitivity [36] . Therefore, understanding the mechanisms leading to HRD and how they might change during prior therapies is important to predict outcomes with PARPi. ARIEL2 is an international, open-label, 2-part, phase 2 study assessing the safety and efficacy of rucaparib as active treatment in patients with relapsed HGOC. Part 1 enrolled patients with platinum-sensitive disease; clinical results and molecular data from this portion were published [17] , [25] , [37] , [38] . Part 2 enrolled patients who had received three to four prior chemotherapies, including patients with platinum-sensitive or platinum-resistant/refractory disease. Here we present clinical results from Part 2 and post hoc exploratory biomarker analyses using the rich dataset of archival tissue samples and screening biopsies required from patients in both Parts 1 and 2. Part 2 efficacy and safety Between October 2013 and August 2016, 491 patients were enrolled and received rucaparib in ARIEL2 (Part 1, n = 204; Part 2, n = 287; Supplementary Fig. S1 ). 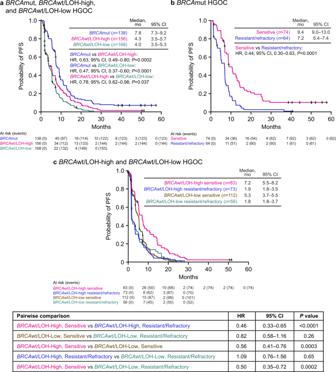Fig. 1: PFS by molecular subgroup and platinum-sensitivity status. aPFS in patients withBRCAmut (blue),BRCAwt/LOH-high (magenta), andBRCAwt/LOH-low (teal) HGOC.bPFS in patients withBRCAmut HGOC that are platinum resistant/refractory (blue) or platinum sensitive (magenta).cPFS in patients withBRCAwt/LOH-high HGOC that are platinum resistant/refractory (blue) or platinum sensitive (magenta) and PFS in patients withBRCAwt/LOH-low HGOC that are platinum resistant/refractory (teal) or platinum sensitive (brown).Pvalues were computed using a Cox proportional hazard model. The interaction between molecular subgroup and platinum status was also tested in the Cox proportional hazard model and found to be significant (P< 0.05).BRCABRCA1orBRCA2, CI confidence interval, HGOC high-grade ovarian carcinoma, HR hazard ratio, LOH loss of heterozygosity, mut mutated, PFS progression-free survival, wt wild type. Baseline demographics and disease characteristics are presented in Table 1 and Supplementary Table S1 . The protocol-prespecified primary endpoints classified patients’ HGOC into one of three HRD groups ( BRCA -mutant [ BRCA mut], BRCA wt/LOH-high, and BRCA wt/LOH-low) using mutations and genome-wide LOH estimates provided by targeted panel NGS of neoplastic tissue (Online Methods) [24] . Among heavily pretreated patients in Part 2, confirmed objective response rates (ORR), the study’s primary endpoint, were 31.0% (95% confidence interval [CI], 21.3–42.0), 6.8% (95% CI, 2.3–15.3), and 5.6% (95% CI, 2.1–11.8), respectively, in patients with BRCA mut, BRCA wt/LOH-high, and BRCA wt/LOH-low HGOC (Supplementary Table S2 ), with durable responses seen across HRD subgroups (Supplementary Fig. S2a ). Data from secondary efficacy endpoints, including ORR by Response Evaluation Criteria In Solid Tumors version 1.1 (RECIST)/Gynecological Cancer InterGroup (GCIG) cancer antigen 125 (CA-125) criteria, progression-free survival (PFS), and overall survival are presented in Supplementary Table S2 and Supplementary Fig. S2b, c . Table 1 Select baseline demographics and disease characteristics. Full size table The toxicity profile of rucaparib in the heavily pretreated patients in Part 2 (Supplementary Tables S3 – S5 ) was consistent with that previously reported in patients with HGOC [7] , [37] , [39] . Molecular subgroup profiling across Parts 1 and 2 Taking advantage of the large sample size with varying degree of platinum sensitivity and number of prior treatments, we analyzed the association between molecular characteristics and clinical outcomes across both parts of ARIEL2 to identify molecular mechanisms resulting in rucaparib sensitivity and resistance. Molecular analyses were used to characterize HGOC based on mutation, methylation, and molecular subgroup status. In these post hoc analyses, molecular subgroups were determined using a 16% LOH cutoff for LOH-high in the BRCA wt subgroup; this refined cutoff was validated within ARIEL2 Part 1 (ref. [40] ) and was prospectively tested in the maintenance setting in ARIEL3 (NCT01968213) [7] . To define the BRCA mut subgroup comprehensively, we utilized both available local testing data and an updated BRCA missense mutation classifier to reclassify the HGOC from 14 patients as BRCA mut, beyond those initially identified by targeted NGS (Supplementary Fig. S3 , Online Methods). In total, 138 HGOC were classified as BRCA mut, 156 were BRCA wt/LOH-high, 168 were BRCA wt/LOH-low, and 29 were BRCA wt/LOH-unclassified. Efficacy based on molecular subgroup and platinum status PFS and ORR differed significantly among molecular subgroups. Patients with BRCA mut HGOC had superior outcomes, with a median PFS of 7.8 months and ORR of 45.7% (95% CI, 37.2–54.3). In contrast, among patients with BRCA wt/LOH-high and BRCA wt/LOH-low HGOC, median PFS was 4.3 months and 4.0 months and ORR was 16.7% (95% CI, 11.2–23.5) and 7.7% (95% CI, 4.2–12.9), respectively (Figs. 1a and 2 and Supplementary Table S6 ). Fig. 1: PFS by molecular subgroup and platinum-sensitivity status. a PFS in patients with BRCA mut (blue), BRCA wt/LOH-high (magenta), and BRCA wt/LOH-low (teal) HGOC. b PFS in patients with BRCA mut HGOC that are platinum resistant/refractory (blue) or platinum sensitive (magenta). c PFS in patients with BRCA wt/LOH-high HGOC that are platinum resistant/refractory (blue) or platinum sensitive (magenta) and PFS in patients with BRCA wt/LOH-low HGOC that are platinum resistant/refractory (teal) or platinum sensitive (brown). P values were computed using a Cox proportional hazard model. The interaction between molecular subgroup and platinum status was also tested in the Cox proportional hazard model and found to be significant ( P < 0.05). BRCA BRCA1 or BRCA2 , CI confidence interval, HGOC high-grade ovarian carcinoma, HR hazard ratio, LOH loss of heterozygosity, mut mutated, PFS progression-free survival, wt wild type. Full size image Fig. 2: ORR based on post hoc molecular subgroups and baseline clinical characteristics. Data are plotted as ORR (dots) with the corresponding two-sided 95% CI (error bars) based on the Clopper–Pearson method. BRCA BRCA1 or BRCA2 , CI confidence interval, HRR homologous recombination repair, LOH loss of heterozygosity, mut mutated, ORR objective response rate, wt wild type. Full size image We hypothesized that cross-resistance mechanisms that emerge during prior lines of platinum treatment affect rucaparib sensitivity. Among patients with BRCA mut HGOC, those who were sensitive to the most recent line of platinum therapy (platinum-free interval [PFI] >6 months) had a median PFS of 9.4 months and ORR of 64.9% (95% CI, 52.9–75.6), whereas those with platinum-resistant (PFI <6 months) or platinum-refractory (progression on prior platinum) disease performed significantly worse, with a median PFS of 7.2 months (hazard ratio [HR], 0.44; 95% CI, 0.30–0.63; P < 0.0001) and ORR of 23.4% (95% CI, 13.8–35.7; P < 0.0001, Fisher’s exact test) (Figs. 1b and 2 and Supplementary Table S6 ). Among patients with BRCA wt HGOC, the LOH-high, platinum-sensitive subgroup performed better (median PFS, 7.2 months; ORR, 27.7% [95% CI, 18.4–38.6]) than the LOH-high, platinum-resistant/refractory subgroup (median PFS, 1.9 months [HR, 0.46; 95% CI, 0.33–0.65]; ORR, 4.1% [95% CI, 0.9–11.5]) and the LOH-low subgroups regardless of platinum status (Fig. 1c ). Genomic scarring is, therefore, a good predictor of rucaparib sensitivity before the emergence of cross-resistance, while LOH-low HGOC lacks PARPi-sensitizing HRD mechanisms, and therefore shows little rucaparib efficacy even with limited prior platinum exposure. Indeed, rucaparib efficacy in BRCA mut and BRCA wt/LOH-high but not BRCA wt/LOH-low HGOC was better for patients with platinum-sensitive disease who had received one or two prior therapies (Part 1) than those who had three or four prior chemotherapy regimens with predominantly platinum-resistant/refractory disease (Part 2) (Fig. 2 and Supplementary Table S6 ). These observations suggest that platinum sensitivity and fewer lines of prior platinum treatments are both linked to better outcomes on rucaparib in HRD-associated HGOC; this finding is further supported by multivariate analyses that identified platinum status and number of prior chemotherapy regimens as significant predictors for ORR (Supplementary Tables S7 and S8 ). Other patient demographics and baseline disease characteristics (age, body mass index, race, Eastern Cooperative Oncology Group performance status, type of ovarian cancer) also tested in multivariate analysis were not identified as significant predictors for response. HRD-associated genetic events leading to rucaparib sensitivity In view of the association between BRCA mutation status and PARPi response [7] , [37] , we examined the relationship between rucaparib response and HRR gene mutation status. Deleterious germline or somatic BRCA mutations were detected in HGOC from 28% of patients (138/491; n = 89 BRCA1 , n = 49 BRCA2 ). Consistent with prior analyses of rucaparib treatment in patients with BRCAmut HGOC, similar ORRs were observed between patients with HGOC associated with germline or somatic BRCA mutations (48.2% [95% CI, 37.3–59.3] and 45.5% [30.4–61.2]; Fig. 2 ). All somatic BRCA mutations were present at similar variant allele fractions to concurrent TP53 mutations, consistent with a driver mutation, and no subclonal somatic BRCA mutations were identified. BRCA reversion mutations restoring the open reading frame were enriched in patients with platinum-resistant/refractory disease and were associated with poor responses to rucaparib [38] . None of the 10 patients who had a reversion mutation before initiating rucaparib achieved a confirmed response (6 progressive disease [PD]; 4 stable disease [SD]). Reversion mutations accounted for 6/16 (37.5%) of BRCA mut HGOC whose best response on rucaparib was PD. We examined whether alterations in 28 HRR genes beyond BRCA (Supplementary Table S9 ) correlated with rucaparib sensitivity. Patients with BRCA wt HGOC associated with any deleterious HRR gene mutation (36/491; 7.3%) had a median PFS of 5.7 months and ORR of 16.7% (95% CI, 6.4–32.8), which was not different from that of patients with BRCA wt HGOC not associated with an HRR gene mutation (median PFS, 3.7 months [HR, 0.83; 95% CI, 0.58–1.20; P = 0.32]; ORR, 11.7% [95% CI, 8.4–15.7]; Supplementary Fig. S4a , Supplementary Table S10 and Fig. 2 ). Given strong evidence linking mutations in PALB2 , RAD51C , and RAD51D to PARPi sensitivity [17] , [37] , [41] , we examined separately how HGOC harboring mutations in any of these three genes responded. Seven patients had HGOC with a deleterious RAD51C/D mutation ( n = 4 RAD51C , n = 3 RAD51D ), and none had a PALB2 mutation. The response rate among the seven patients with RAD51C/D -mutated HGOC was high (5/7; 71.4%; 95% CI, 29.0–96.3; Fig. 2 ). With the exception of one responder with an NBN mutation (Supplementary Table S10 ), all responders with HGOC harboring a non- BRCA HRR gene mutations had a RAD51C or a RAD51D alteration; results from the multivariate analysis also identified RAD51C/D mutation as a significant predictor of ORR (Supplementary Tables S7 and S8 ). Median PFS among patients with RAD51C/D -mutated HGOC was similar to that of patients with BRCA mut HGOC (11.0 and 7.8 months, respectively; HR, 1.52; 95% CI, 0.67–3.44; P = 0.32; Supplementary Fig. S4b ). Although 6/7 RAD51C/D -mutated HGOC were platinum sensitive, one patient had platinum-resistant disease and achieved a partial response to rucaparib, with a PFS of 13.0 months. Additionally, 4/7 patients with RAD51C / D- mutated HGOC had received three or more lines of prior chemotherapy regimens, suggesting that as long as cross-resistance is not present, rucaparib can be highly effective in HGOC with RAD51C/D mutations, even in late lines of treatment. HRD-associated epigenetic events leading to rucaparib sensitivity We assessed the presence of both BRCA1 and RAD51C promoter methylation by methylation-specific polymerase chain reaction (MSP) [25] in available biopsies obtained from archival HGOC tissues ( n = 321), and at screening prior to initiating rucaparib ( n = 230). Consistent with published estimates (11–15% for BRCA1 and 1–3% for RAD51C ) [22] , [42] , ARIEL2 methylation frequencies were 16.8% for BRCA1 and 1.6% for RAD51C in archival tissues, and 13.5% for BRCA1 and 2.6% for RAD51C at screening. None of the BRCA mut HGOC included in the MSP analysis ( n = 79) exhibited BRCA1 promoter methylation, suggesting that BRCA mutations and BRCA1 promoter methylation are mutually exclusive HRD mechanisms. Interestingly, we saw no difference in PFS based on either archival or screening methylation status in patients with BRCA wt HGOC, suggesting that the mere presence of methylation at the two promoters is not a biomarker for rucaparib outcomes (Supplementary Fig. S5 ). MSP analysis detects the presence of methylation but does not estimate what fraction of the neoplastic cells is methylated or if all alleles are silenced [25] . To determine the fraction of methylated BRCA1 and RAD51C copies, we employed methylation-sensitive digital droplet polymerase chain reaction (MS-ddPCR). Initial results from Part 1 platinum-sensitive samples analyzed for quantitative BRCA1 methylation have been published [25] . Here, we report MS-ddPCR analysis of all ARIEL2 patients with BRCA1 or RAD51C promoter methylation detectable by MSP in at least one time point or for whom MSP data were inconclusive. Of the 99 samples submitted (56 archival; 43 screening), 82 were identified as methylated or unmethylated by both methods; four samples that were unmethylated by MSP showed very low levels of methylation by MS-ddPCR (all <2%), suggesting that their methylation levels were below the level of detection of MSP. Methylation in two samples was detected by MSP but was not confirmed by MS-ddPCR. The remaining samples analyzed by MS-ddPCR did not have MSP data available. Only two RAD51C methylated cases, as determined by MSP, were available for MS-ddPCR analysis. Quantitative analysis confirmed low (<70%) RAD51C methylation in the screening and archival samples for both; however, due to this small sample size, RAD51C methylated cases were excluded from quantitative methylation analysis. Using a cutoff of 70% to define high methylation [25] , we observed lower BRCA1 RNA expression among samples with high BRCA1 methylation compared with unmethylated samples ( P < 0.0001, Wilcoxon rank-sum test) (Supplementary Fig. S6a ). However, samples with low methylation had intermediate BRCA1 expression similar to unmethylated cases ( P = 0.079, Wilcoxon rank-sum test). This analysis is consistent with BRCA1 promoter methylation repressing gene expression, with high and low methylation resulting in different levels of BRCA1 suppression and, therefore, differential impact on HRR activity. 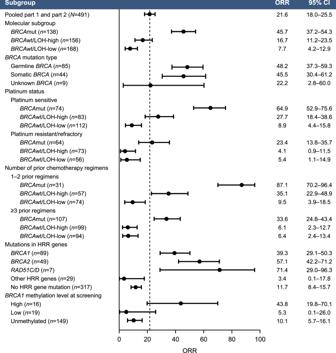Fig. 2: ORR based on post hoc molecular subgroups and baseline clinical characteristics. Data are plotted as ORR (dots) with the corresponding two-sided 95% CI (error bars) based on the Clopper–Pearson method.BRCABRCA1orBRCA2, CI confidence interval, HRR homologous recombination repair, LOH loss of heterozygosity, mut mutated, ORR objective response rate, wt wild type. Although archival BRCA1 methylation levels were not associated with differential PFS with rucaparib treatment (Fig. 3a ), PFS was better in patients with BRCA wt HGOC containing high BRCA1 methylation immediately prior to initiating rucaparib than those with unmethylated or low levels of methylation (Fig. 3b ). Median PFS in patients with high methylation HGOC immediately prior to initiating rucaparib was similar to that of patients with BRCA mut HGOC without reversion mutations (7.8 vs 9.0 months; HR, 0.84; 95% CI, 0.50–1.42; P = 0.52), whereas patients with HGOC with low methylation had a similar median PFS as patients with HGOC with BRCA reversion mutations (2.7 vs 1.8 months; HR, 0.73; 95% CI, 0.33–1.62; P = 0.44) (Supplementary Fig. S6b ). The ORR was 43.8% (95% CI, 19.8–70.1) in patients with high methylation HGOC, 5.3% (95% CI, 0.1–26.0) in patients with low methylation HGOC, and 10.1% (95% CI, 5.7–16.1) in patients with unmethylated HGOC (Fig. 2 ). This difference in response rates indicates that decreased BRCA1 methylation may be an acquired resistance mechanism leading to lower rucaparib efficacy, similar to BRCA reversion mutations. Consistent with these findings, methylation status was identified as a significant predictor of ORR in addition to BRCA and RAD51C/D mutation, in a multivariate analysis (Supplemental Tables S7 and S8 ). Fig. 3: High BRCA1 methylation levels at screening are associated with better outcomes. a Kaplan–Meier plot showing PFS in ARIEL2 patients with BRCA wt HGOC having high (magenta), low (blue), or no methylation (unmethylated, teal) in archival biopsy. b Kaplan–Meier plot showing PFS in ARIEL2 patients with BRCA wt HGOC having high (magenta), low (blue), or no methylation (unmethylated, green) in screening biopsy. P values in panels a and b are based on Cox proportional hazard model. c Methylation status at screening as compared to the archival sample, platinum status, and best response to rucaparib of 17 HGOC with high BRCA1 methylation levels in the archival sample and an available matched screening biopsy; numbers indicate number prior lines of chemotherapy treatment; P values are based on a two-sided Fisher’s exact test testing the proportion of patients with platinum status of sensitive and best response of partial response between HGOC that maintained methylation vs decrease or loss of methylation. BRCA BRCA1 or BRCA2 , CI confidence interval, HGOC high-grade ovarian carcinoma, HR hazard ratio, NA not applicable, PFS progression-free survival, wt wild type. Full size image To examine whether a decrease in methylation correlates with resistance to prior therapies and poor response to rucaparib, we focused on patients with BRCA wt HGOC whose archival samples showed high methylation and who had a matched screening biopsy prior to rucaparib treatment ( n = 17) (Fig. 3c ). HGOCs that maintained high methylation across archival and screening biopsies were enriched for platinum-sensitive disease (6/8), while those with a decrease or loss in methylation were predominantly platinum resistant/refractory (8/9) ( P = 0.015, Fisher’s exact test). Loss/decrease of methylation was also associated with higher number (≥3) of prior lines of chemotherapy treatment ( P = 0.029, Fisher’s exact test; Fig. 3c ). The ORR among the eight patients with HGOC that maintained high methylation was 38%, whereas no responses were observed among the nine with HGOC with methylation decrease or loss (Fig. 3c ), indicating that demethylation may be associated with reduced rucaparib efficacy ( P = 0.082, Fisher’s exact test). Although based on a small number of cases, this analysis suggests that methylation plasticity is an important factor in developing cross-resistance to both platinum agents and PARPi via de-repression of BRCA1 expression and reactivation of HRR. BRCA1 methylation, both high and low, is highly enriched in BRCA wt/LOH-high HGOC compared with other molecular subgroups (Supplementary Table S11 ; P < 0.0001, Chi-square test), confirming an association between methylation and accumulation of genome scars [43] . In ARIEL2, 14% of BRCA wt/LOH-high HGOC (13/94) had high BRCA1 methylation at screening, and 18% (17/94) had low BRCA1 methylation. Outcomes in the two groups were vastly different with ORRs of 46.2% (95% CI, 19.2–74.9) and 5.9% (95% CI, 0.1–28.7; P = 0.025, Fisher’s exact test) in patients with BRCA wt/LOH-high HGOC with high vs low screening methylation, respectively, and median PFS of 9.3 vs 3.3 months (HR, 0.44; 95% CI, 0.21–0.92; P = 0.015). Thus, acquired resistance by demethylation before initiating rucaparib may account for a substantial fraction of PARPi resistance among BRCA wt/LOH-high HGOC, a population expected to be PARPi responsive. Non-HRR gene alterations may modulate response to rucaparib Apart from the HRR pathway, alterations in other pathways may also affect rucaparib response. Mutation and copy number data for 315 genes based on targeted carcinoma NGS were available for 484 of 491 patients. The genetic and epigenetic alterations of HGOC from patients who achieved a confirmed complete or partial response ( n = 103) and those whose best response was PD ( n = 136) are shown in Fig. 4 ; patients who achieved a best response of SD are summarized in Supplementary Fig. S7 . Genes and pathways commonly altered in ovarian cancer were included. TP53 was the most frequently mutated gene (92.8%), consistent with published data [22] , [44] . We also observed frequent alterations in genes involved in non-HRR DNA repair, cell cycle regulation, PI3K/AKT signaling, RAS pathway, and receptor tyrosine kinase signaling. Fig. 4: Genetic and epigenetic alteration landscape of HGOC with confirmed best response of CR/PR (left) or PD (right). Methylation levels shown are at screening. *Short variant include nonsense, missense, frameshift, and splice site alterations. All reported alterations are deleterious or likely deleterious. BRCA BRCA1 or BRCA2 , CR complete response, HGOC high-grade ovarian carcinoma, HRR homologous recombination repair, LOH loss of heterozygosity, mut mutated, PD progressive disease, PR partial response, RTK receptor tyrosine kinase, wt wild type. Full size image Although events in most non-HRR genes are individually rare and did not show significantly different alteration rates between responders and nonresponders, a few interesting observations can be noted. CCNE1 amplification was mutually exclusive with both BRCA mutations, as previously reported [22] , [45] , and BRCA1 methylation. KRAS and NRAS amplifications were enriched among BRCA wt HGOC with PD (14/120, 11.7%); in contrast, no amplification was identified in BRCA wt responders (0/43, P = 0.023, Fisher’s exact test), suggesting that dysregulated RAS signaling may lead to poorer outcomes in BRCA wt HGOC. Several patients ( n = 14) had a KRAS , NRAS , or BRAF activating mutation in the absence of a TP53 mutation, a genetic profile associated with low-grade serous carcinoma, mucinous carcinoma, and mesonephric-like adenocarcinoma [46] , [47] , [48] . A blinded pathology re-review confirmed the presence of non-high-grade serous or non-grade 2/3 endometrioid histologies in 11 of the 14 cases, while all cancers with KRAS , NRAS , or BRAF mutations and a TP53 alteration ( n = 7) were confirmed to be high-grade serous (Supplementary Table S12 and Supplementary Fig. S8 ). Eleven of 12 cancers with KRAS , NRAS , or BRAF activating mutations in TP53 wild-type background that could be classified into molecular subgroups were LOH-low, consistent with the observation that low grade and mesonephric-like histologies are not driven by HRD [49] . Although none of the 14 patients achieved a clinical response to rucaparib, indicating that PARPi are not likely to be active in these rare histologies, some experienced PFS longer than 200 days, an observation that may be indicative of slower overall tumor growth [47] , [50] . Amplification and overexpression in CCNE1 /cell cycle and AKT pathway genes have been previously associated with platinum resistance [42] , [51] . Among platinum-resistant/refractory patients in ARIEL2, patients with BRCA wt HGOC and alterations (predominantly via copy number change) either in the AKT1/2/3 genes or cell cycle pathway at screening had poorer PFS outcomes compared with other patients with BRCA wt HGOC (AKT: HR, 0.45; 95% CI, 0.24–0.85; P = 0.013; cell cycle: HR, 0.66; 95% CI, 0.44–1.00; P = 0.050; Supplementary Fig. S9 ), consistent with the hypothesis that certain platinum resistance mechanisms may modulate responses to other DNA-damaging agents, including PARPi. ARIEL2 assessed the safety and efficacy of rucaparib in an unselected HGOC population. Platinum sensitivity was a strong clinical predictor of rucaparib response in this PARPi-naïve population, especially in the BRCA mut and BRCA wt/LOH-high molecular subgroups. As HRD is a common mechanism leading to both platinum and PARPi sensitivity [1] , this finding suggests that cross-resistance mechanisms arising during platinum therapies also impact responses to PARPi. Here, we describe HRD mechanisms leading to both platinum and rucaparib sensitivity ( BRCA mutation, RAD51C/D alterations, and high BRCA1 promoter methylation) and summarize two important cross-resistance mechanisms: BRCA reversion mutations, which we have previously shown [38] , and loss of BRCA1 methylation described here for the first time using archival and screening clinical specimens. Other cross-resistance mechanisms to PARPi have been previously proposed, including BRCA1 alternative splicing [52] , 53BP1 loss [53] , [54] , increased expression of BRCA hypomorphs [55] , [56] , [57] , and ABCB1 gene fusions [42] , [58] . These mechanisms may also play a role in ARIEL2 but were not assessed here due to insufficient patient samples. Alterations in RAD51C and RAD51D correlated with meaningful clinical activity of rucaparib similar to that of BRCA mut HGOC. Therefore, we propose utilizing panels incorporating RAD51C/D when considering targeted therapies. Importantly, we previously showed that reversion mutations also occur in RAD51C/D as a resistance mechanism [17] , supporting their essential role in generating synthetic lethality with PARPi. The effect of mutations in other HRR genes on rucaparib sensitivity remains unclear given the low relative frequency of each gene in the ARIEL2 cohort. Although it has been hypothesized that ATM mutations are correlated with sensitivity to PARP inhibition, in a recent phase 3 trial, there was no survival benefit seen for patients with prostate cancer associated with ATM mutations who were treated with olaparib vs androgen-receptor targeted therapy (HR, 0.93; 95% CI, 0.53–1.75) [59] . In ARIEL2, no responses were observed among five patients with HGOC harboring an ATM mutation. However, three of these patients had platinum-resistant/refractory disease, and only one of the remaining two was evaluable for response. Therefore, with the limited data, the impact of ATM on rucaparib sensitivity in HGOC remains inconclusive. Through quantitative MS-ddPCR assessment of BRCA1 methylation in archival and screening biopsies, we show that high-level methylation of the BRCA1 promoter is a strong biomarker of rucaparib sensitivity. Patients with carcinomas harboring this modification or a RAD51C/D mutation had PFS similar to that of patients with BRCA mut HGOC treated with rucaparib, even after cases with BRCA reversion mutations are removed from comparison (Fig. 5 ). Further supporting this finding, each of these characteristics (methylation status, BRCA mutation, or RAD51C/D mutation) were identified as a significant predictor for ORR in multivariate analysis. Given strong preclinical data linking BRCA1 promoter methylation to HRD, and platinum and PARPi sensitivity [23] , [24] , the previous lack of definitive clinical evidence associating BRCA1 methylation and therapy response has been perplexing [60] , [61] . The TNT trial (NCT00532727) found no association between BRCA1 methylation and response to carboplatin vs docetaxel in patients with triple-negative breast cancer [26] . Discrepancies between these findings and our own may have both biological and technical explanations. First, most studies analyze methylation in samples obtained at diagnosis, thus missing methylation loss that may have occurred since sample collection. Second, previous studies only report the binary presence or absence of BRCA1 promoter methylation without considering the levels of methylation observed. All BRCA1 alleles likely need to be methylated to establish complete gene silencing and subsequent HRD [26] . Importantly, we show that methylation should be quantitatively assessed immediately prior to treatment to ensure high enough levels to result in sufficient promoter silencing, especially in later-line settings. Fig. 5: High BRCA1 methylation at pretreatment or the presence of a RAD51C/D mutation result in similar PFS as the presence of BRCA mutations. PFS of patients with BRCA mut HGOCs, excluding cases with reversion mutations (blue), patients with HGOCs harboring a RAD51C/D mutation or high methylation at pretreatment (magenta), and all other patients with known mutation and methylation status, including cases with reversion mutations (teal). P values were computed using a Cox proportional hazard model. BRCA BRCA1 or BRCA2 , CI confidence interval, HGOC high-grade ovarian carcinoma, HR hazard ratio, mut mutated, PFS progression-free survival. Full size image Relying on genomic scarring as evidence of HRD in later lines of treatment poses significant disadvantages. Once established, genomic scars persist and do not provide a real-time predictor of sensitivity after multiple treatment lines. In the platinum-sensitive ARIEL2 Part 1 cases, high LOH was associated with a higher ORR among BRCA wt HGOC. But among the more heavily pretreated Part 2 patients, high LOH did not predict rucaparib sensitivity. Notably, all carcinomas with acquired platinum resistance (i.e., BRCA reversion mutation and BRCA1 promoter demethylation) remained LOH-high. Thus, accumulation of genomic scarring is an irreversible process, persisting even as cancers re-acquire functional HRR. In the QUADRA trial of the PARPi niraparib after three lines of therapy, which used the myChoice HRD test to determine HRD status, BRCA mut HGOC were included in the HRD group, driving much of the 15% ORR [62] . When only considering the BRCA wt cases in QUADRA, HRD was associated with a higher ORR only for platinum-sensitive disease (20% vs 4% for non-HRD) and was not predictive for platinum-resistant cases (2.4% vs 3% non-HRD), similar to our findings. Therefore, although stratifying BRCA wt HGOC for PARPi treatment based on evidence of accumulated genomic scarring is useful early in the disease course, these tests lose utility in platinum-resistant/refractory cases. We also examined alterations in non-HRR pathways that may indirectly modulate response to rucaparib. Cell cycle gene alterations, including amplifications of cyclin E, cyclin D, and CDK4/6 genes and deletions in the cell cycle inhibitors CDKN2A/B and CDKN1B , were common in BRCA wt HGOC in ARIEL2 and have been associated with platinum resistance [22] , [63] . AKT signaling has also been linked to platinum resistance, and AKT inhibition appears to reverse resistance in certain models [64] . In ARIEL2, platinum-resistant/refractory BRCA wt HGOC with alterations in the cell cycle pathway and the AKT1/2/3 genes showed poorer outcomes on rucaparib, implying that these pathways may be relevant to responses to multiple DNA-damaging agents. Further in vitro and in vivo studies would be essential to confirm these clinical observations, describe the mechanistic connections between these pathways and PARPi, and determine if combination therapies with PARPi and cell cycle or AKT inhibitors may be beneficial for certain late-stage HGOC patients. Most of the cancers with KRAS , NRAS , or BRAF activating mutations in the absence of a TP53 mutation were subsequently found to be non-HGOC, and the lack of response to rucaparib in these cancers indicates the importance of confirming histological subtype when these mutations are detected. Overall, our analysis highlights significant overlap between molecular mechanisms resulting in platinum and PARPi sensitivity and the extent of cross-resistance that exists between these two drug classes. In addition to BRCA mutations, RAD51C / D mutations and high-level BRCA1 promoter methylation are strong predictors of sensitivity to a PARPi. Given its general tolerability and efficacy, especially in patients with BRCA mut and BRCA wt/LOH-high HGOC, and data supporting the use of PARPi as maintenance following primary therapy [8] , [9] , [10] , [65] , we propose that administration of rucaparib, as active treatment, should be considered in earlier lines of therapy, before the emergence of platinum resistance. Such an approach would increase the likelihood of patients experiencing significant clinical benefit while maintaining the improved quality of life associated with targeted vs systemic therapy. Study design and participants ARIEL2 (CO-338-017; NCT01891344) was an international, multicenter, two-part, phase 2 open-label study conducted across 64 sites in Australia, Canada, France, Spain, the United Kingdom, and the United States. The study design and clinical results from Part 1 were published previously [37] . In ARIEL2, eligible patients were aged 18 years or older with histologically confirmed, relapsed, high-grade serous or Grade 2 or Grade 3 endometroid epithelial ovarian, fallopian tube, or primary peritoneal cancer. Patients were required to have measurable disease according to RECIST, an Eastern Cooperative Oncology Group Performance Status of 0 or 1, and adequate organ function. Part 1 enrolled patients with relapsed HGOC who had received at least one prior platinum-based regimen and had platinum-sensitive disease (disease progression ≥6 months after last platinum). Part 2 enrolled patients with relapsed HGOC who had received three to four prior chemotherapies and had a treatment-free interval of more than 6 months following first-line chemotherapy. Patients in Part 2 could be platinum sensitive, platinum resistant (disease progression <6 months after last platinum, with best response other than PD), or platinum refractory (best response of PD on last platinum with progression-free interval <2 months). Both Part 1 and Part 2 enrolled patients regardless of their HRD status, with the exception that Part 1 had a cap on the number of patients with a known germline BRCA mutation ( n = 15) allowed, in order to enrich for the BRCA wt population. Patients were ineligible if they previously received a PARPi in either the treatment setting or as a maintenance therapy, had an active second malignancy, had central nervous system metastases, or received anticancer therapy 14 days or fewer before receiving their first dose of rucaparib. The study was approved by national or local institutional review boards, as appropriate at each site (see Supplementary Information for full list), and was carried out in accordance with the Declaration of Helsinki and Good Clinical Practice Guidelines of the International Conference on Harmonization. Patients provided written informed consent before participation. Procedures Patients were treated with oral rucaparib at 600 mg twice daily until disease progression, unacceptable toxicity, or death. Supportive care (e.g., antiemetics or analgesics for pain control) was permitted at the investigator’s discretion. Treatment interruptions and dose reductions (in decrements of 120 mg formulation in Part 1 and 100 mg in Part 2) were permitted if a patient had a grade 3 or greater adverse event. Treatment was discontinued if a dose interruption occurred for more than 14 consecutive days (longer dose interruptions were permitted with sponsor approval). Tumor response was assessed by the investigators using RECIST, with computed tomography scans at screening and every 8 weeks (±4 days) during treatment and after treatment for patients who discontinued for any reason other than disease progression. Patients who had been on study at least 18 months could have the frequency of disease assessment decreased to every 16 weeks (±2 days). Assessment continued until confirmed disease progression, death, start of subsequent treatment, or loss to follow-up. Serum CA-125 measures were taken at screening, day 1 of each cycle, and the end of treatment, or when clinically indicated. Hematology, serum chemistry, and safety assessments were done at screening, day 1 and day 15 of cycle 1, and day 1 of any subsequent cycles. Adverse events were classified in accordance with the Medical Dictionary for Drug Regulatory Activities classification system version 19.1 and graded for severity in accordance with the National Cancer Institute’s Common Terminology Criteria for Adverse Event version 4.03 ( https://nciterms.nci.nih.gov/ncitbrowser/start.jsf ). Part 1 patients were treated and followed up until disease progression, death, or discontinuation of treatment due to other reasons. Part 2 patients were followed for survival, subsequent therapy, and secondary malignancy every 12 weeks until death, loss to follow-up, withdrawal of consent from study, or study closure, whichever happened first. Molecular subgroup classification Biomarker analysis was performed following the REMARK (Reporting Recommendations for Tumor Marker Prognostic Studies) guidelines [66] . A known HRR gene mutation was not required for enrollment in ARIEL2. Patients were required to have adequate formalin-fixed paraffin-embedded (FFPE) archival tumor tissue available and to have undergone a pretreatment (screening) biopsy (optional in patients with HGOC having a known deleterious germline BRCA mutation in Part 2). For the ARIEL2 Part 1 and Part 2 prespecified analyses, tumor BRCA status was determined centrally using the FoundationOne TM NGS assay (Supplementary Fig. S3 ) [37] , [67] . Local BRCA test results were collected when available (Supplementary Fig. S3 ). For our post hoc analysis of the pooled ARIEL2 patient population, we classified a patient as BRCA mut if a deleterious BRCA alteration was detected by either central tumor testing or local testing (Supplementary Fig. S3 ). The majority of BRCA alterations that were detected by local testing but not by tissue testing were large rearrangements, known to be challenging to detect by NGS. FoundationOne TM was also used to calculate the percentage of genomic LOH in archival and screening biopsies and to identify alterations in genes other than BRCA [37] , [67] . To classify BRCA wt patients into LOH-high and LOH-low subgroups, we used a prespecified cutoff of 14% for patients in Part 1 and a prespecified cutoff of 18% for patients in Part 2 (Supplementary Fig. S3 ). For the post hoc, exploratory molecular subgroup analyses, both the local and central test information for BRCA was utilized. For BRCA wt, we utilized an optimized cutoff of 16%, which was shown to be the optimal cutoff in ARIEL2 Part 1 (ref. [40] ) and was prospectively evaluated in the phase 3 ARIEL3 study (Supplementary Fig. S3 ) [7] . BRCA1 and BRCA2 germline/somatic status was determined by a combination of methods. Blood samples from all ARIEL2 Part 1 BRCA mut samples and a subset of ARIEL2 Part 2 BRCA mut cases ( n = 74) were analyzed using the BROCA homologous recombination sequencing assay (University of Washington, Seattle WA, USA). Any alteration detected by FoundationOne™ NGS but not BROCA was considered somatic. The remainder of the samples were assigned germline/somatic status based on local testing data provided by the study sites ( n = 29) or computational inference method using the targeted NGS data ( n = 26) [68] . Computational inference was not attempted for samples with tumor purity >80%; those samples were listed as Unknown. Nine BRCA mut cases remained with unknown germline/somatic status. Agreement between germline/somatic status determined through germline sequencing (BROCA and local testing) and the computational inference method was very high for samples that had both data available ( n = 67, 95.5% agreement, kappa = 0.88, P < 0.0001, Cohen’s Kappa statistics). HRR gene mutation subgroup was based on alterations in the genes listed in Supplementary Table S6 . Germline/somatic status for ARIEL2 Part 1 non- BRCA HRR genes was determined by the BROCA homologous recombination sequencing assay (University of Washington, Seattle, WA, USA). Any alteration detected by FoundationOne™ NGS but not BROCA was considered somatic. BRCA wt ARIEL2 Part 2 samples were not analyzed by central germline testing and germline/somatic status for these cases was determined by computational inference as described above [68] . The same computational approach was used to determine zygosity for all non- BRCA HRR gene alterations [68] . The detection of BRCA reversion mutations has been described in detail previously [38] . In short, for reversion mutations present in cell-free DNA (cfDNA), plasma samples collected from ARIEL2 patients were analyzed using the Guardant360 (ref. [69] ) or FoundationACT [70] cfDNA assays. Central tumor tissue NGS data were also re-analyzed to determine if reversion mutations were present. BRCA reversion mutations were defined as: (i) a base substitution that changed a nonsense mutation to a missense mutation, (ii) an insertion/deletion that restored the ORF, or (iii) a larger intragenic deletion that deleted the primary deleterious mutation. Reversion mutations were detected in 10/112 (8.9%) BRCA mut HGOC pretreatment samples: nine by Guardant360 plasma analysis (eight previously described [38] and one identified in post-publication analysis) and one by central tumor tissue NGS analysis. Patients were classified as having a cell cycle pathway alteration if an alteration in any of the following genes was detected in their screening cancer sample: CCNE1 , CCND1 , CCND2 , CCND3 , CDKN2A , CDKN2B , CDKN1B , CDK4 , or CDK6 . Patients were classified as having an AKT alteration if they had an alteration in AKT1 , AKT2 , or AKT3 in their screening cancer sample. Amplifications reported were high-copy gains (CN > 5). 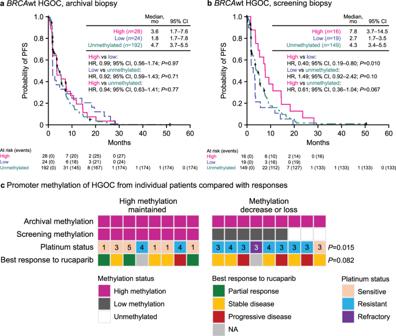Fig. 3: HighBRCA1methylation levels at screening are associated with better outcomes. aKaplan–Meier plot showing PFS in ARIEL2 patients withBRCAwt HGOC having high (magenta), low (blue), or no methylation (unmethylated, teal) in archival biopsy.bKaplan–Meier plot showing PFS in ARIEL2 patients withBRCAwt HGOC having high (magenta), low (blue), or no methylation (unmethylated, green) in screening biopsy.Pvalues in panelsaandbare based on Cox proportional hazard model.cMethylation status at screening as compared to the archival sample, platinum status, and best response to rucaparib of 17 HGOC with highBRCA1methylation levels in the archival sample and an available matched screening biopsy; numbers indicate number prior lines of chemotherapy treatment;Pvalues are based on a two-sided Fisher’s exact test testing the proportion of patients with platinum status of sensitive and best response of partial response between HGOC that maintained methylation vs decrease or loss of methylation.BRCABRCA1orBRCA2, CI confidence interval, HGOC high-grade ovarian carcinoma, HR hazard ratio, NA not applicable, PFS progression-free survival, wt wild type. Methylation analysis The presence of methylation at the BRCA1 and RAD51C promoters was detected using MSP, as previously described [37] . In summary five 10 μm sections of FFPE tissue were deparaffinized, rehydrated, and digested with Proteinase K (Zymo Research, Irvine, CA, USA) overnight and bisulfite conversion of 10 μL of supernatant was performed in duplicates using the EZ DNA Methylation-Direct kit (Zymo Research). Following bisulfite conversion, the samples underwent desulfonation and cleanup, and 2 μL of bisulfite-converted DNA was evaluated with MSP for BRCA1 and RAD51C using primers listed in Supplementary Table S13 . Quantification of BRCA1 and RAD51C methylation levels in HGOC from ARIEL2 Part 1 and Part 2 patients was performed by quantitative MS-ddPCR methodology as previously described [25] : DNA extracted from FFPE-preserved tissue sections was bisulfite converted using the EZ DNA Methylation-Lightning kit (Zymo Research). BRCA1 primers were designed for a 72 bp amplicon in the untranslated region (UTR) (Supplementary Table S13 ). RAD51C methylation, primers were designed for a 142 bp amplicon in the RAD51C UTR. Minor groove binder probes hybridizing to the fully unmethylated (2′-chloro-7′phenyl-1,4-dichloro-6-carboxyfluorescein [VIC] labeled) and the fully methylated sequences (6-carboxyfluorescein [FAM] labeled) were used. The ddPCR was performed on the Bio-Rad QX-200 system. Methylation frequencies determined by MS-ddPCR were normalized to neoplastic purity and BRCA1/RAD51C copy number estimates using the following formula: RM × (CN × TP + (100 − TP) × 2)/(TP × CN)/100, where RM is the raw fraction methylated copies detected, TP is the tumor purity, and CN is the BRCA1 copy number [25] . The tumor purity and copy number were estimated based on the targeted NGS data [68] . Patient samples were classified as having high or low methylation levels based on a predefined cutoff of 70% [25] . In the absence of contradicting MS-ddPCR data, biopsies with 0% BRCA1 promoter methylation by MS-ddPCR, or ones determined to be unmethylated by MSP, were labeled as unmethylated. BRCA1 expression analysis For a subset of the samples analyzed for BRCA1 promoter methylation status, we assessed the BRCA1 RNA expression levels by NanoString [71] . Pathology analysis and histology reclassification For all patients, hematoxylin and eosin (H&E) staining was performed following standard procedures on archival and/or screening biopsy tissue corresponding to the tissue that was submitted for central NGS testing. The H&E slides for the patients harboring activating mutations in the KRAS / NRAS / BRAF genes were re-reviewed by gynecologic pathologists (J.A.E. and D.I.L. ), and a consensus diagnosis was rendered. At time of re-review, the pathologists were blinded to the genomic findings for these patients. Both archival and screening tissue H&E slides were available for at least two patients each for mesonephric-like carcinomas, low-grade serous carcinomas, and endometrioid adenocarcinomas, and the reclassification was confirmed in both samples. Representative fields were selected to describe features concidered for reclassification. Statistical analysis All analyses were performed using the safety population, which included all patients who received at least one dose of rucaparib. The primary endpoint in Part 1 was PFS by predefined HRD subgroups. PFS was defined as the number of days from the first dose of study drug to disease progression by RECIST, as determined by the investigator, or death due to any cause, whichever occurred first. Patients without a documented event of progression were censored on the date of their last adequate cancer assessment (i.e., radiologic assessment) or the date of the first dose of the study drug if no cancer assessments were performed. In Part 2, the primary endpoint was ORR, defined as the proportion of patients achieving a best response of complete or partial response according to RECIST as assessed by the investigator by predefined HRD subgroups. Secondary endpoints included the proportion of patients achieving an objective response (according to RECIST and GCIG CA-125 criteria), duration of response (according to RECIST), and overall survival. Response endpoints were summarized with frequencies and percentage using Clopper–Pearson methodology to calculate 95% CIs. Rates of response were compared with pair-wise comparison using Fisher’s exact test. The response (partial or complete response) by RECIST needed to be confirmed by a second assessment after at least 4 weeks. Duration of confirmed response (complete or partial response) was calculated from the initial date a response was detected to the first date of PD. Patients without a documented event of progression were censored on the date of their last adequate cancer assessment (i.e., radiologic assessment) or date of response if no cancer assessments were performed. Overall survival was defined as the number of days from the date of first dose of study drug to the date of death (due to any cause). Patients without a known date of death were censored on the date the patient was last known to be alive. Duration of response, PFS, and overall survival were summarized with Kaplan–Meier methodology, including median estimates and 95% CIs using log–log distribution. In addition, a Cox proportional hazard model was used to summarize these endpoints and make comparisons between molecular subgroups. Here, we also present post hoc exploratory molecular biomarker analyses of PFS and ORR outcomes in order to further explore clinical benefit. Most of the post hoc analyses are based on univariate comparisons. In addition, a stepwise multivariate logistics regression model was used to identify predictors of confirmed response (PR or CR) using baseline and molecular characteristic variables as predictors in the model (Supplementary Tables S7 and S8 ). 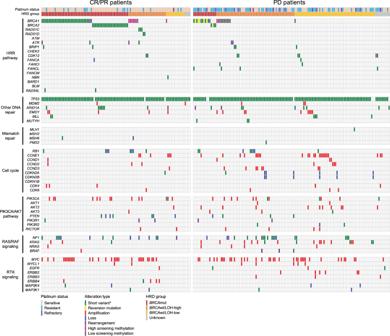Fig. 4: Genetic and epigenetic alteration landscape of HGOC with confirmed best response of CR/PR (left) or PD (right). Methylation levels shown are at screening. *Short variant include nonsense, missense, frameshift, and splice site alterations. All reported alterations are deleterious or likely deleterious.BRCABRCA1orBRCA2, CR complete response, HGOC high-grade ovarian carcinoma, HRR homologous recombination repair, LOH loss of heterozygosity, mut mutated, PD progressive disease, PR partial response, RTK receptor tyrosine kinase, wt wild type. 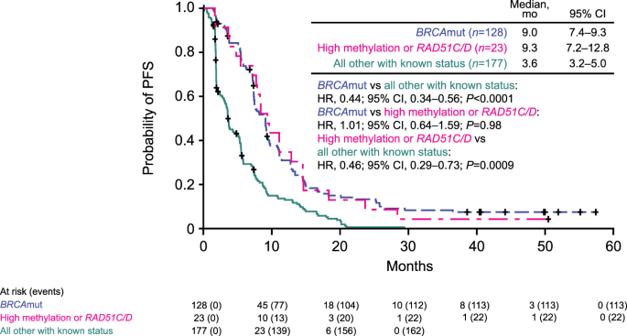Fig. 5: HighBRCA1methylation at pretreatment or the presence of aRAD51C/Dmutation result in similar PFS as the presence ofBRCAmutations. PFS of patients withBRCAmut HGOCs, excluding cases with reversion mutations (blue), patients with HGOCs harboring aRAD51C/Dmutation or high methylation at pretreatment (magenta), and all other patients with known mutation and methylation status, including cases with reversion mutations (teal).Pvalues were computed using a Cox proportional hazard model. BRCABRCA1orBRCA2, CI confidence interval, HGOC high-grade ovarian carcinoma, HR hazard ratio, mut mutated, PFS progression-free survival. For all time-to-event analyses, the proportional hazards assumption was assessed visually with log–log plots (Supplementary Fig. S10 ); as the assumption of the model was valid in each instance, we provide HR and 95% CI for these endpoints. All P values for the post hoc exploratory analyses of molecular subgroups are presented for descriptive purposes only. Comparisons of proportions between methylation subgroups were summarized using Fisher’s exact test or chi-square tests; for the analysis of number prior lines of chemotherapy treatment, patients were grouped in 1–2 and ≥3 prior lines subgroups. The distribution of BRCA1 gene expression levels was analyzed using a nonparametric Wilcoxon rank-sum test to compare molecular subgroups. Agreement analyses were performed using non-weighted Cohen’s Kappa statistics. Data analysis was performed using SAS v9.4 (SAS Institute, Cary, NC, USA) and Excel 2016 (Microsoft Corporation, Redmond, WA, USA). Reporting summary Further information on research design is available in the Nature Research Reporting Summary linked to this article.